Emergence of coherence via transverse condensation in a uniform quasi-two-dimensional Bose gas Phase transitions are ubiquitous in our three-dimensional world. By contrast, most conventional transitions do not occur in infinite uniform low-dimensional systems because of the increased role of thermal fluctuations. The crossover between these situations constitutes an important issue, dramatically illustrated by Bose-Einstein condensation: a gas strongly confined along one direction of space may condense along this direction without exhibiting true long-range order in the perpendicular plane. Here we explore transverse condensation for an atomic gas confined in a novel trapping geometry, with a flat in-plane bottom, and we relate it to the onset of an extended (yet of finite-range) in-plane coherence. By quench crossing the transition, we observe topological defects with a mean number satisfying the universal scaling law predicted by Kibble-Zurek mechanism. The approach described can be extended to investigate the topological phase transitions that take place in planar quantum fluids. Bose–Einstein condensation (BEC) is a remarkably simple phase transition that can in principle occur in a fluid even in the absence of interatomic interactions. As a mere result of single-particle statistics, a phase-coherent fraction appears in the fluid, described by a uniform wave-function spanning the whole system. During the last two decades, cold atom experiments have been used to probe many aspects of BEC [1] , [2] , [3] . However, most of these cold atom studies are performed in the presence of a harmonic confinement. BEC becomes in this case a local transition: the condensate forms at the centre of the trap where the density is the largest, and interactions between particles play a dominant role in the equilibrium state of the fluid. In this geometry, the non-homogeneous character of the gas makes it difficult to address some important features of BEC, such as the existence of long-range phase coherence. The recent achievement of a three-dimensional (3D) Bose gas undergoing BEC in a box-like potential [4] , [5] constitutes an important step forward, realizing the text-book paradigm of an extended and uniform coherent matter wave. When turning to low-dimensional (low-D) systems, subtle effects emerge because of the entangled roles of Bose statistics and thermal fluctuations. First, in an infinite low-D ideal gas, no BEC is expected at non-zero temperature, because of the modification of the single-particle density of states with respect to the 3D case [6] . In other words, the phase coherence between two points tends to zero when their distance increases, contrary to the 3D situation. Second, Bose statistics can play a key role in the dimensional crossover between the 3D situation and a low-D one, by facilitating the freezing of some directions of space. Consider the uniform two-dimensional (2D) case obtained by imposing a tight harmonic trapping potential (frequency ν z ) along the third direction z . The transverse condensation phenomenon [7] , [8] , [9] allows one to reach an effective 2D situation even in the ‘thermally unfrozen’ regime, where the quantum hν z is smaller than the thermal energy k B T ( h and k B stand for Planck’s and Boltzmann’s constants). Third, for the 2D case in the presence of interactions between the particles, the situation gets more involved with the possibility of a superfluid, Berezinskii—Kosterlitz—Thouless (BKT) transition [10] , [11] for a large enough phase-space-density, even though the absence of true long-range coherence remains valid [12] , [13] . This superfluid transition has been identified and characterized over the recent years with non-homogeneous, harmonically trapped Bose gases [14] , [15] , [16] , [17] , [18] , [19] , [20] . Another key feature of phase transitions for uniform systems is the time needed to establish the coherence/quasi-coherence over the whole sample. As is well known for critical phenomena [21] , the coherence length and the thermalization time diverge at the transition point, thus limiting the size of the phase-coherent domains that are formed at its crossing. The Kibble-Zurek (KZ) theory [22] , [23] allows one to evaluate the scaling of the domain size with the speed of the crossing. Once the transition has occurred, these domains start merging together. During this coarsening dynamics singularities taking the form of topological defects can be nucleated at their boundaries, with a spatial density directly related to the characteristic domain size. The KZ mechanism has been studied in a variety of experimental systems (see for example, refs 24 , 25 , 26 , 27 , 28 , 29 ), including cold atomic gases [30] , [31] , [32] , [33] , [34] , [35] , [36] . In 2D quantum fluids, the singularities take the form of quantized vortices, that is, points of zero density around which the macroscopic wavefunction of the gas has a ±2 π phase winding. In this paper, we present an experimental realization of a uniform atomic Bose gas in a quasi-2D geometry, addressing both the steady state of the fluid and its quench dynamics. First with the gas in thermal equilibrium, we characterize the threshold for the emergence of an extended phase coherence by two independent methods, respectively, based on the measurement of the atomic velocity distribution and on matter–wave interferences. We show in particular that for the thermally unfrozen case (with ζ = k B T / hν z ), the transverse condensation phenomenon induces an extended in-plane coherence. Second, we explore the quench dynamics of the gas prepared in an initial state such that and observe density holes associated to vortices. We study the relation between the cooling rate and the number of vortices that subsist after a given relaxation time, and we compare our results with the predictions of the KZ theory. Production of uniform gases in quasi-2D geometries We prepare a cold 3D gas of rubidium ( 87 Rb) atoms using standard laser and evaporative cooling techniques. Then we transfer the gas in a trap formed with two orthogonal laser beams at wavelength 532 nm, shorter than the atomic resonance wavelength (780 nm), so that the atoms are attracted towards the regions of low light intensity ( Fig. 1a ). The strong confinement along the z direction (vertical) is provided by a laser beam propagating along the x direction. It is prepared in a Hermite-Gauss mode, with a node in the plane z =0, and provides a harmonic confinement along the z direction with a frequency ν z in the range 350–1,500 Hz. For the confinement in the horizontal xy plane, we realize a box-like potential by placing an intensity mask on the second laser beam path, propagating along the z direction ( Fig. 1b ). Depending on the study to be performed, we can vary the shape (disk, square, double rectangle) and the area (from 200 to 900 μm 2 ) of the region accessible to the gas in the plane. The relevance of our system for the study of 2D physics is ensured by the fact that the size of the ground state along the z direction is very small compared with the in-plane extension . The number of atoms N that can be stored and reliably detected in this trap ranges between 1,000 and 100,000. We adjust the temperature of the gas in the interval T ~10−250 nK by varying the intensity of the beam creating the box potential, taking advantage of evaporative cooling on the edges of this box. The ranges spanned by ν z and T allow us to explore the dimensional crossover between the thermally frozen regime ( ) and the unfrozen one ( ). Examples of in situ images of 2D gases are shown in Fig. 1c–e . 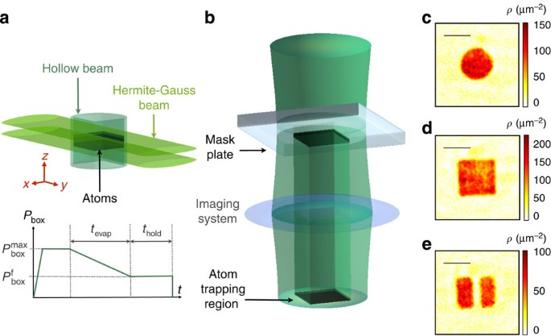Figure 1: Production of uniform Bose gases in quasi-2D geometries. (a) We slice a horizontal sheet from a 3D cold gas of87Rb atoms using a blue detuned laser beam propagating alongxand shaped with an intensity node in thez=0 plane. It creates an adjustable harmonic confinement alongzof frequencyνz=350–1,500 Hz. We superimpose a hollow beam propagating alongzand producing a uniform confinement in thexyplane (seeb). The powerPboxof this beam is ramped up in 10 ms to its maximal valuecorresponding to a potential barrierUbox~kB× 3 μK for the87Rb atoms. After holdingPboxatfor 0.5 s, we lower it linearly to its final valuein a typical time oftevap=2 s and keep it constant for a typicalthold=0.5 s. We varyto adjust the final temperature of the gas via evaporative cooling. (b) The in-plane (xy) confinement is provided by a blue-detuned laser beam shaped by placing a dark intensity mask on its path and imaging it at the position of the atoms. (c–e)In-situdensity distributions of uniform gases trapped in a disk of radiusR=12 μm, a square box of lengthL=30 μm, and two coplanar and parallel rectangular boxes of size 24 × 12 μm2, spaced by 4.5 μm. These distributions are imaged using a high-intensity absorption imaging technique (see Methods). Scale bars, 20 μm. Figure 1: Production of uniform Bose gases in quasi-2D geometries. ( a ) We slice a horizontal sheet from a 3D cold gas of 87 Rb atoms using a blue detuned laser beam propagating along x and shaped with an intensity node in the z =0 plane. It creates an adjustable harmonic confinement along z of frequency ν z =350–1,500 Hz. We superimpose a hollow beam propagating along z and producing a uniform confinement in the xy plane (see b ). The power P box of this beam is ramped up in 10 ms to its maximal value corresponding to a potential barrier U box ~ k B × 3 μK for the 87 Rb atoms. After holding P box at for 0.5 s, we lower it linearly to its final value in a typical time of t evap =2 s and keep it constant for a typical t hold =0.5 s. We vary to adjust the final temperature of the gas via evaporative cooling. ( b ) The in-plane ( xy ) confinement is provided by a blue-detuned laser beam shaped by placing a dark intensity mask on its path and imaging it at the position of the atoms. ( c – e ) In-situ density distributions of uniform gases trapped in a disk of radius R =12 μm, a square box of length L =30 μm, and two coplanar and parallel rectangular boxes of size 24 × 12 μm 2 , spaced by 4.5 μm. These distributions are imaged using a high-intensity absorption imaging technique (see Methods). Scale bars, 20 μm. Full size image Phase coherence in 2D geometries For an ideal gas, an important consequence of Bose-Einstein statistics is to increase the range of phase coherence with respect to the prediction of Boltzmann statistics. Here coherence is characterized by the one-body correlation function , where [resp. ] annihilates (resp. creates) a particle in r , and where the average is taken over the equilibrium state at temperature T . For a gas of particles of mass m described by Boltzmann statistics, G 1 ( r ) is a Gaussian function , where is the thermal wavelength. Consider the particular case of a 2D Bose gas (for example, ). When its phase-space-density becomes significantly larger than 1 ( ρ stands for the 2D spatial density), the structure of G 1 ( r ) changes. In addition to the Gaussian function mentioned above, a broader feature develops, with the characteristic length that increases exponentially with (see ref. 37 and Supplementary Note 1 ) Usually, two main effects amend this simple picture: In a finite system, when the predicted value of becomes comparable to the size L of the gas, one recovers a standard Bose-Einstein condensate, with a macroscopic occupation of the ground state of the box potential [38] . The G 1 function then takes non-zero values for any r ≤ L and the phase coherence extends over the whole area of the gas. In the presence of weak repulsive interactions, the increase of the range of G 1 for is accompanied with a reduction of density fluctuations, with the formation of a ‘quasi-condensate’ or ‘pre-superfluid’ state [15] , [16] , [39] . This state is a medium that can support vortices, which will eventually pair at the superfluid BKT transition for a larger phase-space-density, around for the present strength of interactions [39] . At the transition point, the coherence length diverges and above this point, G 1 ( r ) decays algebraically. Role of the third dimension for in-plane phase coherence When the thermal energy k B T is not negligibly small compared with the energy quantum hν z for the tightly confined dimension, the dynamics associated to this direction brings interesting novel features to the in-plane coherence. First, we note that the function G 1 ( r ) can be written in this case as a sum of contributions of the various states j z of the z motion (see Supplementary Note 1 ). The term with the longest range corresponds to the ground state j z =0, with an expression similar to equation (1), where is replaced by the phase-space-density associated to this state. Now, consider more specifically the unfrozen regime . In this case, one expects that for very dilute gases only a small fraction f 0 of the atoms occupies the j z =0 state; Boltzmann statistics indeed leads to . However, for large total phase-space densities , Bose-Einstein statistics modifies this result through the transverse condensation phenomenon (BEC ⊥ ) [7] : the phase-space-density that can be stored in the excited states j z ≠0 is bounded from above, and can thus become comparable to . This large value of leads to a fast increase of the corresponding range of G 1 ( r ), thus linking the transverse condensation to an extended coherence in the xy plane. This effect plays a central role in our experimental investigation. Phase coherence revealed by velocity distribution imaging To characterize the coherence of the gas, we study the velocity distribution, that is, the Fourier transform of the G 1 ( r ) function. We approach this velocity distribution in the xy plane by performing a 3D time-of-flight (3D ToF): we suddenly switch off the trapping potentials along the three directions of space, let the gas expand for a duration τ , and finally image the gas along the z axis. In such a 3D ToF, the gas first expands very fast along the initially strongly confined direction z . Thanks to this fast density drop, the interparticle interactions play nearly no role during the ToF and the slower evolution in the xy plane is governed essentially by the initial velocity distribution of the atoms. The time-of-flight (ToF) duration τ is chosen so that the size expected for a Boltzmann distribution is at least twice the initial extent of the cloud. Typical examples of ToF images are given in Fig. 2a–f . Whereas for the hottest and less dense configurations, the spatial distribution after ToF has a quasi-pure Gaussian shape, a clear non-Gaussian structure appears for larger N or smaller T . A sharp peak emerges at the centre of the cloud of the ToF picture, signalling an increased occupation of the low-momentum states with respect to Boltzmann statistics, or equivalently a coherence length significantly larger than λ T . 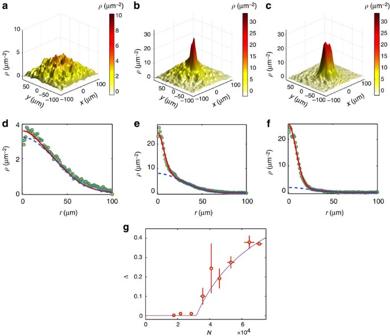Figure 2: Emergence of bimodal velocity distributions. (a–f) Surface density distributionρ(x,y) (first row) and corresponding radial distributions (green symbols) obtained by azimuthal average (second row). The distribution is measured after a 12 ms time-of-flight for a gas initially confined in a square of sizeL=24 μm, with a trapping frequencyνz=365 Hz along thezdirection. The temperaturesTand atom numbersNfor these three realizations area,d: (155 nK, 28,000),b,e: (155 nK, 38,000),c,f: (31 nK, 19,000). The continuous red lines are fits to the data by a function consisting in the sum of two Gaussians corresponding toN1andN2atoms (N=N1+N2). The Gaussian of largest width (N2atoms) is plotted as a blue dashed line. The bimodal parameter Δ=N1/Nequalsa,d: 0.01,b,e: 0.12 andc,f: 0.60. (g) Variation of Δ withNfor a gas in the same initial trapping configuration asa–fand forT=155 nK (red symbols). Error bars are the standard errors of the mean of the binned data set (with four images per point on average). The solid line is a fit to the data by the functionf(N)=(1−(Nc/N)0.6) forN>Nc, andf(N)=0 forN≤Nc, from which we deduceNc(T). HereNc=3.2(1) × 104, where the uncertainty range is obtained by a jackknife resampling method, that is, fitting samples corresponding to a randomly chosen fraction of the global data set. Figure 2: Emergence of bimodal velocity distributions. ( a – f ) Surface density distribution ρ ( x , y ) (first row) and corresponding radial distributions (green symbols) obtained by azimuthal average (second row). The distribution is measured after a 12 ms time-of-flight for a gas initially confined in a square of size L =24 μm, with a trapping frequency ν z =365 Hz along the z direction. The temperatures T and atom numbers N for these three realizations are a , d : (155 nK, 28,000), b , e : (155 nK, 38,000), c , f : (31 nK, 19,000). The continuous red lines are fits to the data by a function consisting in the sum of two Gaussians corresponding to N 1 and N 2 atoms ( N = N 1 + N 2 ). The Gaussian of largest width ( N 2 atoms) is plotted as a blue dashed line. The bimodal parameter Δ= N 1 / N equals a , d : 0.01, b , e : 0.12 and c , f : 0.60. ( g ) Variation of Δ with N for a gas in the same initial trapping configuration as a – f and for T =155 nK (red symbols). Error bars are the standard errors of the mean of the binned data set (with four images per point on average). The solid line is a fit to the data by the function f ( N )=(1−( N c / N ) 0.6 ) for N > N c , and f ( N )=0 for N ≤ N c , from which we deduce N c ( T ). Here N c =3.2(1) × 10 4 , where the uncertainty range is obtained by a jackknife resampling method, that is, fitting samples corresponding to a randomly chosen fraction of the global data set. Full size image In order to analyse this velocity distribution, we chose as a fit function the sum of two Gaussians of independent sizes and amplitudes, containing N 1 and N 2 atoms, respectively (see Fig. 2d–f ). We consider the bimodality parameter Δ= N 1 / N defined as the ratio of the number of atoms N 1 in the sharpest Gaussian to the total atom number N = N 1 + N 2 . A typical example for the variations of Δ with N at a given temperature is shown in Fig. 2g for an initial gas with a square shape (side length L =24 μm). It shows a sharp crossover, with essentially no bimodality ( ) below a critical atom number N c ( T ) and a fast increase of Δ for N > N c ( T ). We extract the value N c ( T ) by fitting the function Δ ∝ (1−( N c / N ) 0.6 ) to the data. We chose this function as it provides a good representation of the predictions for an ideal Bose gas in similar conditions (see Methods). Phase coherence revealed by matter–wave interference Matter–wave interferences between independent atomic or molecular clouds are a powerful tool to monitor the emergence of extended coherence [4] , [14] , [40] , [41] , [42] . To observe these interferences in our uniform setup, we first produced two independent gases of similar density and temperature confined in two coplanar parallel rectangles, separated by a distance of 4.5 μm along the x direction (see Fig. 1e ). Then we suddenly released the box potential providing confinement in the xy plane, while keeping the confinement along the z direction (2D ToF). The latter point ensures that the atoms stay in focus with our imaging system, which allows us to observe interference fringes with a good resolution in the region where the two clouds overlap. A typical interference pattern is shown in Fig. 3a , where the fringes are (roughly) parallel to the y axis, and show some waviness that is linked to the initial phase fluctuations of the two interfering clouds. 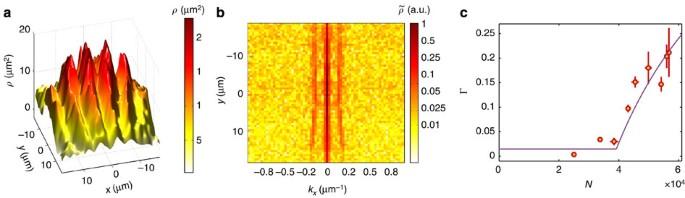Figure 3: Emergence of coherence via matter–wave interference. (a) Example of a density distribution after a 16 ms in-plane expansion of two coplanar clouds initially confined in rectangular boxes of size 24 × 12 μm2, spaced by 4.5 μm (νz=365 Hz). The region of interest considered in our analysis consists of 56 lines and 74 columns (pixel width: 0.52 μm). (b) Amplitude of the 1D Fourier transform of each line of the density distribution. Each lineyshows two characteristic side peaks at ±kp(y) above the background noise, corresponding to the fringes pattern ofa. Here ‹kp›=0.17(2) μm−1. (c) Variation of the average contrast Γ (see text for its definition) for images of gases atT=155 nK. Error bars show the standard errors of the mean of the binned data set (with on average three images per point). The solid line is a fit to the data of the functionf(N) defined asf(N)=bforN≤Ncandf(N)=b+a(1−(Nc/N)0.6) forN>Nc. The parameterbis a constant for a data set with variousTtaken in the same experimental conditions. Here we deduceNc=3.9(2) × 104, where the uncertainty range is obtained by a jackknife resampling method. Figure 3: Emergence of coherence via matter–wave interference. ( a ) Example of a density distribution after a 16 ms in-plane expansion of two coplanar clouds initially confined in rectangular boxes of size 24 × 12 μm 2 , spaced by 4.5 μm ( ν z =365 Hz). The region of interest considered in our analysis consists of 56 lines and 74 columns (pixel width: 0.52 μm). ( b ) Amplitude of the 1D Fourier transform of each line of the density distribution. Each line y shows two characteristic side peaks at ± k p ( y ) above the background noise, corresponding to the fringes pattern of a . Here ‹ k p ›=0.17(2) μm −1 . ( c ) Variation of the average contrast Γ (see text for its definition) for images of gases at T =155 nK. Error bars show the standard errors of the mean of the binned data set (with on average three images per point). The solid line is a fit to the data of the function f ( N ) defined as f ( N )= b for N ≤ N c and f ( N )= b + a (1−( N c / N ) 0.6 ) for N > N c . The parameter b is a constant for a data set with various T taken in the same experimental conditions. Here we deduce N c =3.9(2) × 10 4 , where the uncertainty range is obtained by a jackknife resampling method. Full size image We use these interference patterns to characterize quantitatively the level of coherence of the gases initially confined in the rectangles. For each line y of the pixelized image acquired on the CCD camera, we compute the x -Fourier transform of the spatial density ρ ( x , y ) ( Fig. 3b ). For a given y , this function is peaked at a momentum k p ( y )>0 that may depend (weakly) on the line index y . Then we consider the function that characterizes the correlation of the complex fringe contrast along two lines separated by a distance d Here * denotes the complex conjugation and the average is taken over the lines y that overlap with the initial rectangles. If the initial clouds were two infinite, parallel lines with the same G 1 ( y ), one would have γ ( d )=| G 1 ( d )| 2 (ref. 43 ). Here the non-zero extension of the rectangles along x and their finite initial size along y make it more difficult to provide an analytic relation between γ and the initial G 1 ( r ) of the gases. However, γ ( d ) remains a useful and quantitative tool to characterize the fringe pattern. For a gas described by Boltzmann statistics, the width at 1/ e of G 1 ( r ) is and remains below 1 μm for the temperature range investigated in this work. Since we are interested in the emergence of coherence over a scale that significantly exceeds this value, we use the following average as a diagnosis tool For the parameter Γ to take a value significantly different from 0, one needs a relatively large contrast on each line, and relatively straight fringes over the relevant distances d , so that the phases of the different complex contrasts do not average out. For a given temperature T , the variation of Γ with N shows the same threshold-type behaviour as the bimodality parameter Δ. One example is given in Fig. 3c , from which we infer the threshold value for the atom number N c ( T ) needed to observe interference fringes with a significant contrast. Scaling laws for the emergence of coherence We have plotted in Fig. 4 the ensemble of our results for the threshold value of the total 2D phase-space-density as a function of ζ = k B T / hν z , determined both from the onset of bimodality as in Fig. 2g (closed symbols) or from the onset of visible interference as in Fig. 3c (open symbols). Two trapping configurations have been used along the z direction, ν z =1,460 Hz and ν z =365 Hz. In the first case, the z direction is nearly frozen for the temperatures studied here ( ). In the second one, the z direction is thermally unfrozen ( ). All points approximately fall on a common curve, independent of the shape and the size of the gas: varies approximately linearly with ζ with the fitted slope 1.4 (3) for and approaches a finite value ~4 for . 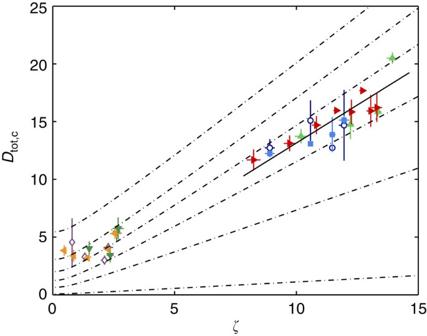Figure 4: Scaling law for the emergence of coherence in a uniform Bose gas in a quasi-2D geometry. Variation of the threshold phase-space-densityfor observing a non-Gaussian velocity distribution (full symbols) and distinct matter–wave interferences (open symbols), as a function of the dimensionless parameterζ=kBT/(hνz). For velocity distribution measurements:νz=365 Hz: disk of radiusR=12 μm (red left triangles), disk ofR=9 μm (light green up triangle), square ofL=24 μm (blue square);νz=1,460 Hz: disk ofR=12 μm (orange right triangles), disk ofR=9 μm (dark green down triangles). For interference measurements:νz=365 Hz: dark blue open circles;νz=1,460 Hz: violet open diamonds. Error bars show the 95% confidence bounds on theNcparameter of the threshold fits to the data sets. The black solid line shows a linear fit to the data forζ>8, leading toDtot, c=1.4(3)ζ. The black dash–dotted lines show contours of identical ratios of the coherence range to the thermal wavelengthλT. The coherence range is evaluated by the value ofrat whichG1(r)=G1(0)/20 (see text) and we plot (in increasingDtotorder) ratios equal to 1, 1.2, 1.5, 2, 3 and 8. Boltzmann prediction corresponds to a ratio of ~0.98. Figure 4: Scaling law for the emergence of coherence in a uniform Bose gas in a quasi-2D geometry. Variation of the threshold phase-space-density for observing a non-Gaussian velocity distribution (full symbols) and distinct matter–wave interferences (open symbols), as a function of the dimensionless parameter ζ = k B T /( hν z ). For velocity distribution measurements: ν z =365 Hz: disk of radius R =12 μm (red left triangles), disk of R =9 μm (light green up triangle), square of L =24 μm (blue square); ν z =1,460 Hz: disk of R =12 μm (orange right triangles), disk of R =9 μm (dark green down triangles). For interference measurements: ν z =365 Hz: dark blue open circles; ν z =1,460 Hz: violet open diamonds. Error bars show the 95% confidence bounds on the N c parameter of the threshold fits to the data sets. The black solid line shows a linear fit to the data for ζ >8, leading to D tot, c =1.4(3) ζ . The black dash–dotted lines show contours of identical ratios of the coherence range to the thermal wavelength λ T . The coherence range is evaluated by the value of r at which G 1 ( r )= G 1 (0)/20 (see text) and we plot (in increasing D tot order) ratios equal to 1, 1.2, 1.5, 2, 3 and 8. Boltzmann prediction corresponds to a ratio of ~0.98. Full size image In the frozen case, a majority of atoms occupy the vibrational ground state j z =0 of the motion along the z direction, so that essentially represents the 2D phase-space-density associated to this single transverse quantum state. Then for , we know from equation (1) and the associated discussion that a broad component arises in G 1 with a characteristic length that increases exponentially with the phase-space-density. The observed onset of extended coherence around can be understood as the place where starts to exceed significantly λ T . The regime around is reminiscent of the presuperfluid state identified in refs 15 , 16 . It is different from the truly superfluid phase, which is expected at a higher phase-space-density ( ) for our parameters [39] . Therefore, the threshold is not associated to a true phase transition, but to a crossover where the spatial coherence of the gas increases rapidly with the control parameter N . For ν z =365 Hz, the gas is in the ‘unfrozen regime’ ( ), which could be naively thought as irrelevant for 2D physics since according to Boltzmann statistics, many vibrational states along z should be significantly populated. However, thanks to the BEC ⊥ phenomenon presented above, a macroscopic fraction of the atoms can accumulate in the j z =0 state. This happens when the total phase-space-density exceeds the threshold for BEC ⊥ (cf. Supplementary Note 1 and Supplementary Fig. 1 ): In the limit ζ →∞, BEC ⊥ corresponds to a phase transition of the same nature as the ideal gas BEC in 3D (see Supplementary Note 1 and Supplementary Fig. 2 ). In the present context of our work, we emphasize that although BEC ⊥ originates from the saturation of the occupation of the excited states along z , it also affects the coherence properties of the gas in the xy plane. In particular when rises from 0 to , the coherence length in xy increases from ~ λ T (the non-degenerate result) to ~ a z , the size of the ground state of the z motion (see Supplementary Note 1 , Supplementary Fig. 3 and Supplementary Table 1 ). This increase can be interpreted by noting that when BEC ⊥ occurs (equation 4), the 3D spatial density in the central plane ( z =0) is equal to , where g s is the polylogarithm of order s and g 3/2 (1)≈2.612 (see Supplementary Note 1 and Supplementary Fig. 4 ). For an infinite uniform 3D Bose gas with this density, a true BEC occurs and the coherence length diverges. Because of the confinement along the z direction, such a divergence cannot occur in the present quasi-2D case. Instead, the coherence length along z is by essence limited to the size a z of the j z =0 state. When the same limitation applies in the transverse plane, giving rise to coherence volumes that are grossly speaking isotropic. When is increased further, the coherence length in the xy plane increases, while remaining limited to a z along the z direction. The results shown in Fig. 4 are in line with this reasoning. For , the emergence of coherence in the xy plane occurs for a total phase-space-density , with a proportionality coefficient α =1.4(3) in good agreement with the prediction π 2 /6≈1.6 of equation (4). We have also plotted in Fig. 4 contour lines characterizing the coherence range in terms of ζ and . Using ideal Bose gas theory, we calculated the one-body coherence function G 1 ( r ) and determined the distance r f over which it decreases by a given factor f with respect to G 1 (0). We chose the value f =20 to explore the long tail that develops in G 1 when phase coherence emerges. The contour lines shown in Fig. 4 correspond to given values of r 20 / λ T ; they should not be considered as fits to the data, but as an indication of a coherence significantly larger than the one obtained from Boltzmann statistics (for which r 20 ≈ λ T ). The fact that the threshold phase-space densities follow quite accurately these contour lines validates the choice of tools (non-Gaussian velocity distributions, matter–wave interferences) to characterize the onset of coherence. Observation of topological defects From now on we use the weak trap along z ( ν z =365 Hz) so that the onset of extended coherence is obtained thanks to the transverse condensation phenomenon. We are interested in the regime of strongly degenerate, interacting gases, which is obtained by pushing the evaporation down to a point where the residual thermal energy k B T becomes lower than the chemical potential μ (see Methods for the calculation of μ in this regime). The final box potential is ~ k B × 40 nK, leading to an estimated temperature of ~10 nK, whereas the final density (~50 μm −2 ) leads to μ≈ k B × 14 nK. In these conditions, for most realizations of the experiment, defects are present in the gas. They appear as randomly located density holes after a short 3D ToF ( Fig. 5a,b ), with a number fluctuating between 0 and 5. To identify the nature of these defects, we have performed a statistical analysis of their size and contrast, as a function of their location and of the ToF duration τ ( Fig. 5c,d ). For a given τ , all observed holes have similar sizes and contrasts. The core size increases approximately linearly with τ , with a nearly 100% contrast. This favours the interpretation of these density holes as single vortices, for which the 2π phase winding around the core provides a topological protection during the ToF. This would be the case neither for vortex–antivortex pairs nor phonons, for which one would expect large fluctuations in the defect sizes and lower contrasts. 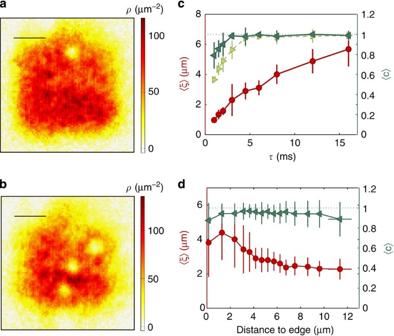Figure 5: Observation of vortices. (a,b) Examples of density distributions (scale bars, 10 μm) after a 3D ToF ofτ=4.5 ms for a gas initially confined in a square of sizeL=30 μm (νz=365 Hz). The two examples show, respectively, one (a) and three (b) holes of high contrast, corresponding to topologically protected expanding vortex cores. We fit each density hole by a hyperbolic tangent dip convoluted by a Gaussian of waistw=1 μm accounting for imaging imperfections (see Methods). (c) Evolution of the average sizeξ(red circles, left labels) and contrastc(green triangles, right labels) of density holes with the expansion durationτ. No holes are visible forms. Red circles and dark green left triangles are results from a fit accounting for imaging imperfections, whereas light green right triangles show contrast resulting from a fit without a convolution by a Gaussian. (d) Variation of the hole sizeξ(red circles, left labels) and contrastc(green triangles, right labels) with the distance to the nearest edge of the box (same configuration asa,b: ToF ofτ=4.5 ms for a gas in a square ofL=30 μm). For a distance larger than ~4 μm,ξandcare approximately independent from the vortex location. The average values incare taken over all holes independent of their positions. One point inc(resp.d) corresponds to 15 (resp. 70) vortex fits. Error bars show standard deviations of the binned data set. Figure 5: Observation of vortices. ( a , b ) Examples of density distributions (scale bars, 10 μm) after a 3D ToF of τ =4.5 ms for a gas initially confined in a square of size L =30 μm ( ν z =365 Hz). The two examples show, respectively, one ( a ) and three ( b ) holes of high contrast, corresponding to topologically protected expanding vortex cores. We fit each density hole by a hyperbolic tangent dip convoluted by a Gaussian of waist w =1 μm accounting for imaging imperfections (see Methods). ( c ) Evolution of the average size ξ (red circles, left labels) and contrast c (green triangles, right labels) of density holes with the expansion duration τ . No holes are visible for ms. Red circles and dark green left triangles are results from a fit accounting for imaging imperfections, whereas light green right triangles show contrast resulting from a fit without a convolution by a Gaussian. ( d ) Variation of the hole size ξ (red circles, left labels) and contrast c (green triangles, right labels) with the distance to the nearest edge of the box (same configuration as a , b : ToF of τ =4.5 ms for a gas in a square of L =30 μm). For a distance larger than ~4 μm, ξ and c are approximately independent from the vortex location. The average values in c are taken over all holes independent of their positions. One point in c (resp. d ) corresponds to 15 (resp. 70) vortex fits. Error bars show standard deviations of the binned data set. Full size image Dynamical origin of the topological defects In principle, the vortices observed in the gas could be due to steady-state thermal fluctuations. BKT theory indeed predicts that vortices should be present in an interacting 2D Bose gas around the superfluid transition point [11] . Such ‘thermal’ vortices have been observed in non-homogeneous atomic gases, either interferometrically [14] or as density holes in the trap region corresponding to the critical region [20] . However, for the large and uniform phase-space densities that we obtain at the end of the cooling process ( ), ref. 44 predicts a vanishingly small probability of occurrence for such thermal excitations. This supports a dynamical origin for the observed defects. To investigate further this interpretation, we can vary the two times that characterize the evolution of the gas, the duration of evaporation t evap and the hold duration after evaporation t hold (see Fig. 1a ). For the results presented in this section, we fixed t hold =500 ms and studied the evolution of the average vortex number N v as a function of t evap . The corresponding data, given in Fig. 6a , show a decrease of N v with t evap , passing from N v ≈1 for t evap =50 ms to N v ≈0.3 for t evap =250 ms. For longer evaporation times, N v remains approximately constant around 0.35(5). 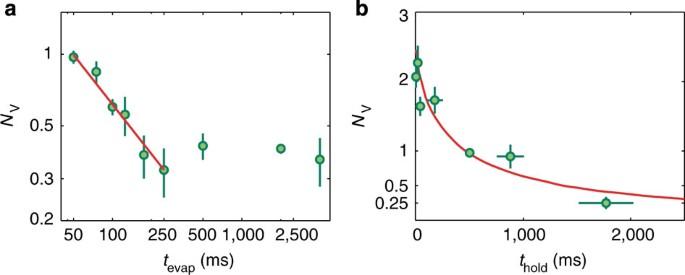Figure 6: Dynamics of vortex nucleation. (a) Circle symbols: evolution of the mean vortex numberNvwith the quench timetevap(fixedthold=500 ms) for a gas initially confined in a square of sizeL=30 μm (νz=365 Hz) and observed after a 3D ToF ofτ=4.5 ms. The number of images per point ranges from 37 to 233, with a mean of 90. We restrict totevap≥50 ms to ensure that local thermal equilibrium is reached at any time during the evaporation ramp58. Red line: fit of a power-law decay to the short time data (tevap≤250 ms), giving the exponentd=0.69(17). The uncertainty range ondis the 95% confidence bounds of a linear fit to the evolution of log(Nv) with log(tevap). For longer quench times, the mean vortex numbers are compatible with a plateau atNv=0.35(5). (b) Circle symbols: evolution of the mean vortex numberNvwith the hold timethold(fixedtevap=50 ms) in the same experimental configuration asa. The number of images per point ranges from 24 to 181, with a mean of 59. In both figures, error bars are obtained from a bootstrapping approach. Red line: results from a model describing the evolution of an initial number of vorticesNv,0=2.5(2) in the presence of a phenomenological damping coefficient47. The inferred superfluid fraction is 0.94(2). Confidence ranges on these parameters are obtained from aχ2analysis. Figure 6: Dynamics of vortex nucleation. ( a ) Circle symbols: evolution of the mean vortex number N v with the quench time t evap (fixed t hold =500 ms) for a gas initially confined in a square of size L =30 μm ( ν z =365 Hz) and observed after a 3D ToF of τ =4.5 ms. The number of images per point ranges from 37 to 233, with a mean of 90. We restrict to t evap ≥50 ms to ensure that local thermal equilibrium is reached at any time during the evaporation ramp [58] . Red line: fit of a power-law decay to the short time data ( t evap ≤250 ms), giving the exponent d =0.69(17). The uncertainty range on d is the 95% confidence bounds of a linear fit to the evolution of log( N v ) with log( t evap ). For longer quench times, the mean vortex numbers are compatible with a plateau at N v =0.35(5). ( b ) Circle symbols: evolution of the mean vortex number N v with the hold time t hold (fixed t evap =50 ms) in the same experimental configuration as a . The number of images per point ranges from 24 to 181, with a mean of 59. In both figures, error bars are obtained from a bootstrapping approach. Red line: results from a model describing the evolution of an initial number of vortices N v,0 =2.5(2) in the presence of a phenomenological damping coefficient [47] . The inferred superfluid fraction is 0.94(2). Confidence ranges on these parameters are obtained from a χ 2 analysis. Full size image The decrease of N v with t evap suggests that the observed vortices are nucleated via a KZ type mechanism [22] , [23] , [45] , occurring when the transition to the phase coherent regime is crossed. However, applying the KZ formalism to our setup is not straightforward. In a weakly interacting, homogeneous 3D Bose gas, BEC occurs when the 3D phase-space-density reaches the critical value g 3/2 (1). For our quasi-2D geometry, transverse condensation occurs when the 3D phase-space-density in the central plane z =0 reaches this value. At the transition point, the KZ formalism relates the size of phase-coherent domains to the cooling speed . For fast cooling, KZ theory predicts domain sizes for a 3D fluid that are smaller than or comparable to the thickness a z of the lowest vibrational state along z ; it can thus provide a good description of our system. For a slower cooling, coherent domains much larger than a z would be expected in 3D at the transition point. The 2D nature of our gas leads in this case to a reduction of the in-plane correlation length. In the slow cooling regime, we thus expect to find an excess of topological defects with respect to the KZ prediction for standard 3D BEC. More explicitly we expect for fast cooling, hence short t evap , a power-law decay with an exponent d given by the KZ formalism for 3D BEC. The fit of this function to the measured variation of N v for t evap ≤250 ms leads to d =0.69(17) (see Fig. 6a ). This is in good agreement with the prediction d =2/3 obtained from the critical exponents of the so-called ‘F model’ [21] , which is believed to describe the universality class of the 3D BEC phenomenon. For comparison, the prediction for a pure mean-field transition, d =1/2, is notably lower than our result. For longer t evap , the above described excess of vortices due to the quasi-2D geometry should translate in a weakening of the decrease of N v with t evap . The non-zero plateau observed in Fig. 6a for t evap ≥250 ms may be the signature of such a weakening. Other mechanisms could also play a role in the nucleation of vortices for slow cooling. For example, because of the box potential residual rugosity, the gas could condense into several independent patches of fixed geometry, which would merge later during the evaporation ramp and stochastically form vortices with a constant probability. Lifetime of the topological defects The variation of the number of vortices N v with the hold time t hold allows one to study the fate of vortices that have been nucleated during the evaporation. We show in Fig. 6b the results obtained when fixing the evaporation to a short value t evap =50 ms. We observe a decay of N v with the hold time, from N v =2.3 initially to 0.3 at long t hold (2 s). To interpret this decay, we modelled the dynamics of the vortices in the gas with two ingredients: first the conservative motion of a vortex in the velocity field created by the other vortices, including the vortex images from the boundaries of the box potential [46] ; second the dissipation induced by the scattering of thermal excitations by the vortices, which we describe phenomenologically by a friction force that is proportional to the non-superfluid fraction of atoms in the gas [47] . During this motion, a vortex annihilates when it reaches the edge of the trap or encounters another vortex of opposite charge. The numerical solution of this model leads to a non-exponential decay of the average number of vortices, with details that depend on the initial number of vortices and their locations. Assuming a uniform random distribution of vortices at the end of the evaporation, we have compared the predictions of this model to our data. It gives the following values of the two adjustable parameters of the model, the initial number of vortices N v,0 =2.5(2) and the superfluid fraction 0.94(2); the corresponding prediction is plotted as a continuous line in Fig. 6b . We note that at short t hold , the images of the clouds are quite fuzzy, probably because of non-thermal phononic excitations produced (in addition to vortices) by the evaporation ramp. The difficulty to precisely count vortices in this case leads to fluctuations of N v at short t hold as visible in Fig. 6b . The choice t hold =500 ms in Fig. 6a was made accordingly. The finite lifetime of the vortices in our sample points to a general issue that one faces in the experimental studies on the KZ mechanism. In principle, the KZ formalism gives a prediction on the state of the system just after crossing the critical point. Experimentally we observe the system at a later stage, at a moment when the various domains have merged, and we detect the topological defects formed from this merging. In spite of their robustness, the number of vortices is not strictly conserved after the crossing of the transition and its decrease depends on their initial positions. A precise comparison between our results and KZ theory should take this evolution into account, for example, using stochastic mean-field methods [48] , [49] , [50] , [51] . Using a box-like potential created by light, we developed a setup that allowed us to investigate the quantum properties of atomic gases in a uniform quasi-2D configuration. Thanks to the precise control of atom number and temperature, we characterized the regime for which phase coherence emerges in the fluid. The uniform character of the gas allowed us to disentangle the effects of ideal gas statistics for in-plane motion, the notion of transverse condensation along the strongly confined direction and the role of interactions. This is to be contrasted with previous studies that were performed in the presence of a harmonic confinement in the plane, where these different phenomena could be simultaneously present in the non-homogeneous atomic cloud. For the case of a weakly interacting gas considered here, our observations highlight the importance of Bose statistics in the emergence of extended phase coherence. This coherence is already significant for phase-space densities , well below the value required either for the superfluid BKT transition or for the full BEC in the ground state of the box (see Supplementary Note 2 and Supplementary Fig. 5 ). For our parameters, the latter transitions are expected around the same phase-space-density (~8–10) meaning that when the superfluid criterion is met, the coherence length set by Bose statistics is comparable to the box size. By cooling the gas further, we entered the regime where interactions dominate over thermal fluctuations. This allowed us to visualize with a very good contrast the topological defects (vortices) that are created during the formation of the macroscopic matter-wave, as a result of a KZ type mechanism. Here we focused on the relation between the vortex number and the cooling rate. Further investigations could include correlation studies on vortex positions, which can shed light on their nucleation process and their subsequent evolution [52] . Our work motivates future research in the direction of strongly interacting 2D gases [19] , for which the order of the various transitions could be interchanged. In particular, the critical for the BKT transition should decrease, and reach ultimately the universal value of the ‘superfluid jump’, (ref. 53 ). In this case, the emergence of extended coherence in the 2D gas would be essentially driven by the interactions. Indeed, once the superfluid transition is crossed, the one-body correlation function is expected to decay very slowly, G 1 ( r ) ∝ r − α , with α <1/4. It would be interesting to revisit the statistics of formation of quench-induced topological defects in this case, for which significant deviations to the KZ power-law scaling have been predicted [54] , [55] . Characterization of the box-like potential We create the box-like potential in the xy plane using a laser beam that is blue-detuned with respect to the 87 Rb resonance. At the position of the atomic sample, we image a dark mask placed on the path of the laser beam. This mask is realized by a metallic deposit on a wedged, anti-reflective-coated glass plate. We characterize the box-like character of the resulting trap in two ways. First, the flatness of the domain where the atoms are confined is characterized by the root mean square intensity fluctuations of the inner dark region of the beam profile. The resulting variations of the dipolar potential are δU / U box ~3%, where U box is the potential height on the edges of the box. The ratio δU / k B T varies from ~40% at the loading temperature to ~10% at the end of the evaporative cooling (ramp of U box , see below). In particular, it is of ~20% at the transverse condensation point for the configuration in which the vortex data have been acquired. Second, the sharp spatial variation of the potential at the edges of the box-like trapping region is characterized by the exponent α of a power-law fit U ( r ) ∝ r α along with a radial cut. We restrict the fitting domain to the central region where U ( r )< U box /4 and find α ~10–15, depending on the size and the shape of the box. Imaging of the atomic density distribution We measure the atomic density distribution in the xy plane using resonant absorption imaging along z . We use two complementary values for the probe beam intensity I . First, we use a conventional low-intensity technique with I / I sat ≈0.7, where I sat is the saturation intensity of the Rb resonance line, with a probe pulse duration of 20 μs. This procedure enables a reliable detection of low-density atomic clouds, but it is unfaithful for high-density ones, especially in the 2D geometry because of multiple scattering effects between neighbouring atoms [56] . We thus complement it by a high-intensity technique inspired from ref. 57 , in which we apply a short pulse of 4 μs of an intense probe beam with I / I sat ≈40. ToF bimodality measurements (where the cloud is essentially 3D at the moment of detection) were performed with the low-intensity procedure. This was also the case for the matter–wave interference measurements, for which we reached a better fringe visibility in this case. In situ images in Fig. 1 and all data related to vortices (for example, Fig. 5a,b ) in the strongly degenerate gases were taken with high-intensity imaging. We estimate the uncertainty on the atom number to be of 20%. Ideal gas description of trapped atomic samples We consider a gas of N non-interacting bosonic particles confined in a square box of size L in the xy plane, and in a harmonic potential well of frequency ν z along z . The eigenstates of the single-particle Hamiltonian are labelled by three integers j x , j y ≥1, j z ≥0: where a z =( h / mν z ) 1/2 /(2 π ) and χ j is the normalized j th Hermite function. Their energies and occupation factors are where μ<0 is the chemical potential of the gas and N =∑ j n j . The average value of any one-body observable can then be calculated: Interaction energy estimate for weakly interacting gases We estimate the local value of the interaction energy per particle , where a =5.1 nm is the 3D scattering length characterizing s -wave interactions for 87 Rb atoms and ρ (3D) ( r ) the spatial 3D density estimated using the ideal gas description. It is maximal at trap centre r =0. For example, using a typical experimental condition with N =40,000 atoms in a square box of size L =24 μm at T =200 nK, we find a maximal 3D density of ρ (3 D ) (0)=13.8 μm −3 . The mean-field interaction energy for an atom localized at the centre of cloud is then . We note that is negligible compared with k B T and hν z for all atomic configurations corresponding to the onset of an extended phase coherence. In this case, the interactions play a negligible role in the 2D ToF expansion that we use to reveal matter–wave interferences. Temperature calibration All temperatures indicated in the paper are deduced from the value of the box potential, assuming that the evaporation barrier provided by U box sets the thermal equilibrium state of the gas. This hypothesis was tested, and the relation between T and U box calibrated, using atomic assemblies with a negligible interaction energy. For these assemblies, we compared the variance of their velocity distribution Δ v 2 obtained from a ToF measurement to the prediction of equation (8). The calibration obtained from this set of measurements can be empirically written as where the values of the dimensionless parameter η and of the reference temperature T 0 slightly depend on the precise shape of the trap. For the square trap of side 24 μm, we obtain T 0 =191(6) nK and η =3.5(3). The reason for which T saturates when the box potential increases to infinity is due to the residual evaporation along the vertical direction, above the barrier created by the horizontal Hermite–Gauss beam. Power exponent for fitting N c We estimate the behaviour of Δ( N ) at fixed T using Bose law for a ideal gas. We compute from equation (8) the equilibrium velocity distribution Then we estimate the spatial density after a ToF of duration τ (for a disk trap of radius R ) via , where stands for the convolution operator and Θ for the Heaviside function. We fit ρ ( r ) to a double Gaussian and compute the atom fraction in the sharpest Gaussian Δ, similar to the processing of experimental data. To simulate our experimental results, we consider ν z =350 Hz, R =12 μm, τ =14 ms and T varying from 100 to 250 nK. For a given T , we record Δ while varying the total atom number N from 0.06 to 4 times the theoretical critical number for (see Supplementary Note 1 ). We fit Δ( N ) between N min =0.06 N c,th and a varying N max in 1.1–4 N c,th , to f ( N )=(1−( N c / N ) α ) with N c as a free parameter and a fixed α . For all considered T and N max , choosing α =0.6 provides both a good estimate of N c (between 0.93 and 0.99 N c,th ) and a satisfactory fit (average coefficient of determination 0.94). Chemical potential in the degenerate interacting regime To compute the chemical potential μ of highly degenerate interacting gases, we perform a T =0 mean-field analysis. We solve numerically the 3D Gross–Pitaevskii equation in imaginary time using a split-step method, and we obtain the macroscopic ground-state wave-function ψ ( r ). Then we calculate the different energy contributions at T =0—namely the potential energy E pot , the kinetic energy E kin and interaction energy E int —by integrating over space: with ω z =2 πν z . We obtain the value of the chemical potential μ by taking the derivative of the total energy with respect to N and subtracting the single-particle ground-state energy: In the numerical calculation, we typically use time steps of 10 −4 ms and compute the evolution for 10 ms. The 3D grid contains 152 × 152 × 32 voxels, with a voxel size 0.52 × 0.52 × 0.26 μm 3 . Analysis of the density holes created by the vortices We first calculate the normalized density profile , where the average is taken over the set of images with the same ToF duration τ . Then we look for density minima with a significant contrast and size. Finally, for each significant density hole, we select a square region centred on it with a size that is approximately three times larger than the average hole size for this τ . In this region, we fit the function to the normalized density profile, where A 0 accounts for density fluctuations. We also correct for imaging imperfections (finite imaging resolution and finite depth of field) by performing a convolution of the function defined in equation (14) by a Gaussian of width 1 μm, which we determined from a preliminary analysis. How to cite this article: Chomaz, L. et al. Emergence of coherence via transverse condensation in a uniform quasi-two-dimensional Bose gas. Nat. Commun. 6:6162 doi: 10.1038/ncomms7162 (2015).